Gold-like activity copper-like selectivity of heteroatomic transition metal carbides for electrocatalytic carbon dioxide reduction reaction An overarching challenge of the electrochemical carbon dioxide reduction reaction (eCO 2 RR) is finding an earth-abundant, highly active catalyst that selectively produces hydrocarbons at relatively low overpotentials. Here, we report the eCO 2 RR performance of two-dimensional transition metal carbide class of materials. Our results indicate a maximum methane (CH 4 ) current density of −421.63 mA/cm 2 and a CH 4 faradic efficiency of 82.7% ± 2% for di-tungsten carbide (W 2 C) nanoflakes in a hybrid electrolyte of 3 M potassium hydroxide and 2 M choline-chloride. Powered by a triple junction photovoltaic cell, we demonstrate a flow electrolyzer that uses humidified CO 2 to produce CH 4 in a 700-h process under one sun illumination with a CO 2 RR energy efficiency of about 62.3% and a solar-to-fuel efficiency of 20.7%. Density functional theory calculations reveal that dissociation of water, chemisorption of CO 2 and cleavage of the C-O bond—the most energy consuming elementary steps in other catalysts such as copper—become nearly spontaneous at the W 2 C surface. This results in instantaneous formation of adsorbed CO—an important reaction intermediate—and an unlimited source of protons near the tungsten surface sites that are the main reasons for the observed superior activity, selectivity, and small potential. The electrocatalytic carbon dioxide reduction reaction (eCO 2 RR) driven by renewable energy has great potential for the sustainable production of chemicals and fuels at the gigaton scale that can be used any time, any place [1] , [2] , [3] , [4] . It also offers a promising way to store energy in chemical bonds due to having nearly two orders of magnitude higher energy density compared to the most advanced battery technologies [5] . However, reducing CO 2 to value-added chemicals is both costly and slow based on intrinsic thermodynamics and kinetics, making the goal of an effective and feasible process a real challenge [6] , [7] , [8] , [9] . Conventional pure metal catalysts such as gold (Au), palladium (Pd), silver (Ag), and newly developed transition metal dichalcogenides (TMDCs) [8] , [10] , [11] , [12] , [13] , [14] , [15] , [16] , [17] , [18] are known to exhibit high activities for the CO 2 RR in different electrolyte solutions [19] , [20] , [21] , [22] , [23] , [24] , [25] , [26] . However, these catalysts are mainly selective for carbon monoxide (CO), known as an intermediate product [8] , [27] . Other catalysts such as copper (Cu) and Cu-based catalysts have the ability to reduce CO 2 to various chemicals such as methane (CH 4 ), ethylene (C 2 H 4 ), formic acid (HCOOH), methanol (CH 3 OH), and ethanol (C 2 H 5 OH) [28] , [29] , [30] , [31] , [32] , [33] , [34] , [35] , [36] . Despite their good selectivity, these catalysts require high potentials—excess energy—to achieve suitable current densities—reaction rates—impeding their use for effective production of chemicals and fuels [37] , [38] . Therefore, an effective catalyst needs to be developed to selectively produce hydrocarbons at high rates at relatively low potentials. Heteroatomic transition metal carbide (TMC) catalysts, also known as MXenes, have recently received great attention for various electrocatalytic reactions due to their unique structural and electronic properties [39] , [40] , [41] , [42] . In particular, M 2 C (M denotes transition metals) stoichiometry of this class of two-dimensional materials forms layered structures of M-C-M where a plane of carbon atoms is sandwiched between two hexagonal planes of metal atoms. This structure provides a high density of active metal atoms at the surface breaking conventional scaling relationships that limit the electrocatalytic performance of their counterparts such as TMDCs and pure metals [43] . However, there is limited knowledge of their performance and characteristics as eCO 2 RR catalysts under actual experimental conditions. In this work, we investigate the performance of di-tungsten carbide (W 2 C), di-molybdenum carbide (Mo 2 C), diniobium carbide (Nb 2 C), and divanadium carbide (V 2 C) nanoflakes (NFs) as inexpensive, non-precious members of TMCs for eCO 2 RR. Our electrochemical results indicate that W 2 C NFs work remarkably well for eCO 2 RR by achieving a maximum CH 4 formation current density of −421.63 mA/cm 2 and faradaic efficiency of 82.7% ± 2 that are the highest values yet reported. These results suggest a catalytic activity higher than Au, product selectivity similar to Cu in the CO 2 RR for W 2 C NFs. Our DFT calculations also reveal that dissociation of water, chemisorption of CO 2 , and cleavage of the C–O bond, known as the most energy-consuming elementary steps in other catalysts, become nearly spontaneous at the W 2 C surface and are the main reason for the observed superior activity, selectivity, and small overpotential for CH 4 production. The TMC NFs i.e., W 2 C, Mo 2 C, Nb 2 C, and V 2 C were synthesized using a carburization process followed by the liquid exfoliation technique (Supplementary section 1 ) [27] , [44] , [45] . The electrocatalytic performance of TMC NFs with similar crystallite sizes (25.4 ± 5 nm) were then studied in a three-electrode cell and compared with Au and Cu nanoparticles (NPs), conventional catalysts for this reaction, [46] under identical experimental conditions (Supplementary section 2 ). To improve the CO 2 RR performance in competing with hydrogen evolution reaction (HER), we have employed a mixture of 3 M potassium hydroxide (KOH) and 2 M choline chloride (CC) solution (KOH:CC 3 M:2 M) as the electrolyte in this study [47] . The linear sweep voltammetry (LSV) experiments and a real-time product stream analysis show that CO 2 RR on the W 2 C surface starts at a potential of −122.7 mV vs reversible hydrogen electrode (RHE) by producing CO and H 2 and reach maximum CO 2 RR current density ( j CO2RR ) of −548.9 mA/cm 2 at −1.05 V vs RHE (Supplementary Figs. 2 – 4 and Fig. 1a ). As shown in Fig. 1a , j CO2RR of −419.9, −381.9, and −350.8 mA/cm 2 were observed for Mo 2 C, Nb 2 C, and V 2 C NFs, respectively, at this potential (Supplementary section 3 ). However, Au and Cu NPs exhibit a j CO2RR of −208.11 and −89.53 mA/cm 2 at −1.05 V vs RHE (Fig. 1a ). The selectivity analysis also indicates that TMC NFs produce hydrocarbons (i.e., CH 4 , C 2 H 4 , CH 3 OH, and C 2 H 5 OH) at a potential range of −0.45 to −1.05 V vs RHE for W 2 C, Mo 2 C, and Nb 2 C NFs and a potential range of −0.55 to −1.05 V vs RHE for V 2 C NFs where CH 4 is identified as the main product (Supplementary section 3 ). Fig. 1: Electrocatalytic performance of TMCs i.e., W 2 C, Mo 2 C, Nb 2 C, V 2 C NFs in the two-compartment three-electrode electrochemical cell using CO 2 saturated KOH:CC (3 M:2 M) electrolyte. a CO 2 reduction reaction current densities ( j CO2 ) of TMCs compared to Au and Cu NPs at different cathodic potentials (E WE ) under identical experimental condition. b CH 4 formation current densities ( j CH4 ) of TMCs compared to Cu NPs at different potentials (E WE ) under identical experimental condition. 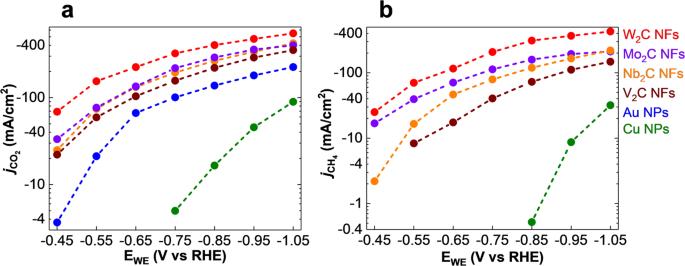Fig. 1: Electrocatalytic performance of TMCs i.e., W2C, Mo2C, Nb2C, V2C NFs in the two-compartment three-electrode electrochemical cell using CO2saturated KOH:CC (3 M:2 M) electrolyte. aCO2reduction reaction current densities (jCO2) of TMCs compared to Au and Cu NPs at different cathodic potentials (EWE) under identical experimental condition.bCH4formation current densities (jCH4) of TMCs compared to Cu NPs at different potentials (EWE) under identical experimental condition. Full size image Figure 1b illustrates CH 4 formation current densities ( j CH4 , mA/cm 2 ) of the TMC NFs compared to Cu NPs, a conventional catalyst for hydrocarbon production. The partial current densities of different products (i.e., H 2 , CO, CH 4 , C 2 H 4 , CH 3 OH, and C 2 H 5 OH) were calculated by multiplying FEs and total current densities at different potentials (Supplementary section 3 and Supplementary Fig. 3 ). As shown in Fig. 1b , a maximum j CH4 of −421.63 mA/cm 2 is obtained for W 2 C NFs at a potential of −1.05 V vs RHE where Nb 2 C NFs, Mo 2 C NFs, and V 2 C NFs show values of −219.16, −211.33, and −147.56 mA/cm 2 , respectively, at this potential. 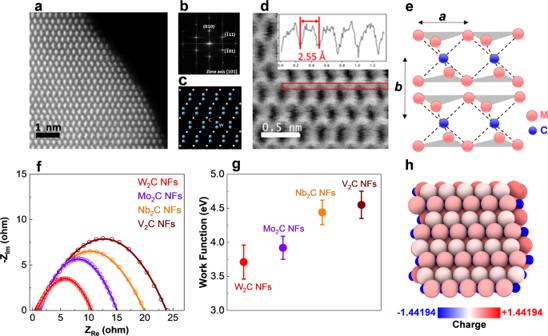Fig. 2: Structural and electrochemical characterization of TMC catalysts. aHigh-angle annular dark-field (HAADF) of W2C NFs in <101> zone axis.bFFT corresponding to the HAADF image of W2C NFs showing the diffraction spots from <101> zone axis.cAtomic model of W2C NFs in <101> zone axis. W atoms are shown as blue and carbon atoms as white spheres.dBright field (BF) of W2C NFs in <101> zone axis. It shows the carbon atomic columns in a red box. The inset is intensity profile across red box region showing the distance between two carbon atoms is 2.55 Å.eSchematic of 1T structure TMCs showing tetragonal symmetry, one layer per repeat unit with octahedral coordination. The transition metal atoms (W, Mo, Nb, and V) are red and the carbon atoms are blue. The lattice constantais in the range of 3.07 to 3.15 Å for synthesized TMCs. The stacking indexbindicates the interlayer spacing which is in the range of 4.53 to 5 Å for studied TMCs.fElectrochemical impedance spectroscopy (EIS) for studied catalysts at a potential of −310 mV vs RHE in the two-compartment three-electrode electrochemical cell using KOH:CC (3 M:2 M) electrolyte.gWork function measurements for synthesized TMCs using ultraviolet photoelectron spectroscopy (UPS) method.hBader charges of W2C NFs indicate that surface W-atoms are contributing significantly to the catalytic activity of the W2C (101) surface. We also compared the CH 4 formation activity of TMCs i.e., W 2 C, Nb 2 C, Mo 2 C, and V 2 C NFs with state-of-the-art catalysts in the literature by calculating their maximum CH 4 formation current densities ( j max.CH4 , Supplementary Table 2 ) [46] , [48] , [49] , [50] , [51] , [52] , [53] , [54] . Supplementary Table 2b indicates that the j max.CH4 of W 2 C NFs is 3.6 and 4.2 times higher than recently studied La 2 CuO 4 (−117 mA/cm 2 at −1.4 V vs RHE) [51] and Cu–N (−100 mA/cm 2 at −1.0 V vs RHE) [48] , respectively. The partial current densities of other hydrocarbon products i.e., C 2 H 4 , CH 3 OH, and C 2 H 5 OH are also shown in Supplementary Fig. 3 (Supplementary section 3 ). To evaluate the intrinsic activity of W 2 C NFs, we measured CH 4 formation turnover frequency (TOF CH4 ) by normalizing its activity to the number of active atoms at the surface using the roughness factor method and compared it with the other catalysts in this study (Supplementary section 5 ). Our calculations indicate a TOF CH4 of 10.42 s −1 at a potential of −1.05 V vs RHE for W 2 C NFs; by comparison, TOF CH4 of 4.54, 3.74, and 2.79 s −1 were calculated for Mo 2 C NFs, Nb 2 C NFs, and V 2 C NFs, respectively. 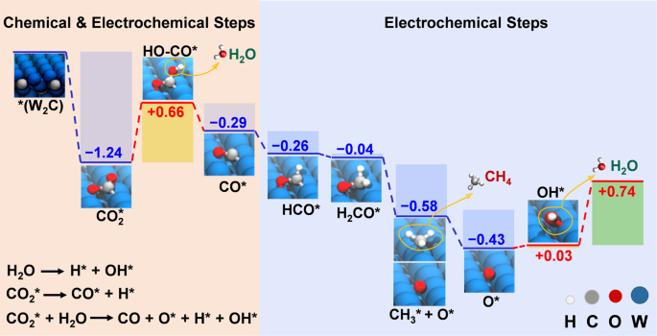Fig. 3: Minimum energy path for the electrochemical CO2conversion into CH4on the surface of W2C NFs. Only electrochemical steps are shown. The parts of the reaction where chemical and electrochemical steps are essential are highlighted by colors. The favorable reactions of key chemical steps are provided (for free energies of these reactions, see TableS9). The intermediates are indicated. Gibbs free energies for reaction at zero potential vs RHE are given in eV. The calculated TOF CH4 of W 2 C NFs at the potential of −1.05 V vs RHE is about two orders of magnitude higher than that of Cu NPs (0.0736 s −1 ) under identical experimental conditions (Supplementary Fig. 7a ). Moreover, total CO 2 RR turnover frequencies (TOF CO2RR ) of 19.09, 19.36, 17.82, and 17.55 s −1 were calculated for W 2 C NFs, Mo 2 C NFs, Nb 2 C NFs, and V 2 C NFs, respectively, where Au NPs and Cu NPs exhibit TOF CO2RR of 4.35 and 0.1956 s −1 , respectively (Supplementary Fig. 7f ). These results suggest the superior CH 4 selectivity of TMC catalysts compared to state-of-the-art catalysts [48] , [49] , [50] , [51] , [54] , [55] , [56] , [57] . Furthermore, we performed a comparative mechanistic study by calculating Tafel slopes for different products to gain insight about the eCO 2 RR mechanism of the TMCs i.e., W 2 C, Mo 2 C, Nb 2 C, and V 2 C NFs in the two-compartment three-electrode electrochemical cell (Supplementary section 6 and Supplementary Fig. 8 ) [58] . Our Tafel plot analyses show that the TMC NFs possess steeper Tafel slopes, and therefore a weaker potential dependence compared with Cu NPs for the formed products (i.e., CO, CH 4 , and C 2 H 4 ) (Supplementary Fig. 8 ) [58] . The Tafel plot analyses suggest a different CO 2 RR mechanism for TMC NFs than that of Cu catalysts where C–O bond scission is the rate-determining step [58] . To gain more insight to the remarkable performance of these catalysts for electrocatalytic CO 2 RR, the structural and physicochemical properties of TMC NFs were characterized at molecular and atomic scales by performing X-ray diffraction (XRD), X-ray photoelectron spectroscopy (XPS), and scanning transmission electron microscopy (STEM) (Supplementary sections 7 – 9 ). At first, we have performed XPS experiments to analyze the surface chemistry of TMC NFs. XPS analysis (Supplementary Fig. 9 ) indicates that our NF samples contain metallic TMCs, with little or no evident surface oxidation. The results show that the chemical composition of the surface, the empirical formula of M 2 C (M: transition metal, C: Carbide), and the oxidation state of +2 for the transition metals i.e., W, Mo, Nb, and V are similar in all synthesized TMCs (Supplementary section 7 ). The lattice structure and crystallite size of the TMC NFs were then studied by performing XRD experiments. The XRD pattern of W 2 C NFs shows a sharp peak at 39.91° along with three pronounced peaks at 34.84°, 38.54°, and 52.65° corresponding to (101), (100), (002), and (102) crystal surfaces of W 2 C, respectively. The XRD spectra of the TMCs show all Bragg peaks of W 2 C, Mo 2 C, Nb 2 C, and V 2 C NFs; verifying their homogenous and pure structures. The XRD results indicate a constant dominant lattice plane of (101) and a similar average crystallite size of 25.4 ± 5 nm for all synthesized TMCs (Supplementary Fig. 10 ) [59] , [60] , [61] . Furthermore, we performed atomic-scale STEM experiments to study surface atom coordination, crystallite sizes, and dominant plane structures of TMC NFs (Supplementary Figs. 11 – 18 ). Figure 2a–d shows STEM results of W 2 C NFs. Figure 2a, b indicate high-angle annular dark-field (HAADF) image and corresponding fast Fourier transforms (FFT) of W 2 C NFs in the <101> zone axis. The atomic models of the <101> zone axis and bright-field (BF) image of W 2 C NFs are represented in Fig. 2c and d , respectively. Figure 2d indicates the carbon atomic columns in the red box and the intensity profile across the red box region showing that the distance between two carbon atoms is 2.55 Å. The STEM results of other TMCs i.e., Mo 2 C, Nb 2 C, and V 2 C NFs are explained in Supplementary section 9 . The STEM and XRD results of synthesized TMC NFs confirm that the structure of these materials is a perfect match with the standard 1T structure, suggesting a tetragonal symmetry and octahedral coordination of the atoms (Fig. 2e ) [43] , [62] . Figure 2e indicates the schematic of 1T structure TMC NFs showing tetragonal symmetry, one layer per repeat unit with octahedral coordination. The lattice constant a is in the range of 3.07 to 3.15 Å for synthesized TMC NFs. The stacking index b indicates the interlayer spacing which is in the range of 4.53 to 5 Å for studied TMCs. As shown in Fig. 2e , 1T atomic coordination provides metal-terminated surface atoms that are known to be favorable binding sites of adsorbed intermediates in eCO 2 RR [43] , [62] . Our atomic and molecular scale structural analyses indicate that the synthesized TMC NFs have fairly similar structural properties e.g., (1T) crystalline structure with a dominant plane of (101), crystallite sizes, and atomic coordination. Fig. 2: Structural and electrochemical characterization of TMC catalysts. a High-angle annular dark-field (HAADF) of W 2 C NFs in <101> zone axis. b FFT corresponding to the HAADF image of W 2 C NFs showing the diffraction spots from <101> zone axis. c Atomic model of W 2 C NFs in <101> zone axis. W atoms are shown as blue and carbon atoms as white spheres. d Bright field (BF) of W 2 C NFs in <101> zone axis. It shows the carbon atomic columns in a red box. The inset is intensity profile across red box region showing the distance between two carbon atoms is 2.55 Å. e Schematic of 1T structure TMCs showing tetragonal symmetry, one layer per repeat unit with octahedral coordination. The transition metal atoms (W, Mo, Nb, and V) are red and the carbon atoms are blue. The lattice constant a is in the range of 3.07 to 3.15 Å for synthesized TMCs. The stacking index b indicates the interlayer spacing which is in the range of 4.53 to 5 Å for studied TMCs. f Electrochemical impedance spectroscopy (EIS) for studied catalysts at a potential of −310 mV vs RHE in the two-compartment three-electrode electrochemical cell using KOH:CC (3 M:2 M) electrolyte. g Work function measurements for synthesized TMCs using ultraviolet photoelectron spectroscopy (UPS) method. h Bader charges of W 2 C NFs indicate that surface W-atoms are contributing significantly to the catalytic activity of the W 2 C (101) surface. Full size image To further discern the difference between the observed electrocatalytic performance of the TMCs, we have studied their electronic properties by performing electrochemical impedance spectroscopy (EIS) (Supplementary section 11 ) and, work function measurements using ultraviolet photoelectron spectroscopy (UPS) (Supplementary section 12 ) [8] . At first, we have employed the EIS experiments to compare the overall electron-transfer properties of the TMC catalysts in the double layer region (Supplementary section 11). To do this, TMC NFs with similar structural and physical properties e.g., sizes, shapes, and mass loadings (0.1 mg/cm 2 ) coated on glass carbon were used as the working electrodes. This results in similar roughness, morphology, intrinsic capacitance, and exposed surface area of the studied samples confirmed by our characterization results (Supplementary sections 5 – 10 ). The EIS experiments have been performed at a potential of −310 mV vs RHE for all TMCs under identical experimental conditions (Supplementary section 11 ). Figure 2f shows the fitted EIS spectra of each TMC catalyst using Randles circuit model, indicating a smaller charge transfer resistance (R ct ) for W 2 C NFs (~17 ohm) compared to the other TMCs, i.e., Mo 2 C NFs (~25 ohm), Nb 2 C NFs (~33 ohm), and V 2 C NFs (~38 ohm) [63] . The UPS method also was used to compare the surface work function of TMCs (Fig. 2g ). The results indicate a lower work function for W 2 C NFs (0.2 to 0.84 eV) compared to Mo 2 C NFs (3.92 eV), Nb 2 C NFs (4.44 eV), and V 2 C NFs (4.55 eV). The charge transfer resistance obtained by EIS experiments and the surface work function value measured by UPS experiments suggests the superior activity of W 2 C NFs compared to other TMCs in this study i.e., Mo 2 C, Nb 2 C, and V 2 C NFs. In addition to our experimental observations, we have performed density functional theory (DFT) calculations to gain more insight to the electronic and catalytic properties of M 2 C compounds. The aim is to address the enhanced activity and selectivity of these TMCs and to explore both electrochemical (i.e., driven) and chemical (i.e., favorable or spontaneous) processes that distinguish them from other catalysts, such as Au and Cu. With respect to activity, the electronic density of states (DOS) indicate that transition metal d states dominate at the Fermi level of these TMCs, much more so than elemental Au, another high activity catalyst. Bader charge calculations indicate that metal atoms at the TMC surface are significantly more reduced compared to the bulk atoms (Fig. 2h and Supplementary Fig. 24 ). These results indicate the increased availability of electrons at metal-rich TMC surfaces, which may increase the catalytic activity of TMC NFs. With respect to the increased selectivity of TMC NFs, especially for CH 4 production, we have explored the CO 2 RR pathway on the W 2 C (101) surface in detail by using DFT calculations. Focusing initially on electrochemical processes, we employed the computational hydrogen electrode (CHE) model [64] , [65] , [66] (Supplementary Tables 7 – 10 ) to explore the stepwise electronic reduction and protonation of adsorbed species in the low molecular coverage limit. The lowest free energy pathway to produce CH 4 with only electrochemical steps is shown in Fig. 3 and Supplementary Fig. 27 . The same steps with only a slight adjustment for experimental Faradaic efficiencies at the potential for optimal CH 4 production is provided in Supplementary Fig. 26 ). Fig. 3: Minimum energy path for the electrochemical CO 2 conversion into CH 4 on the surface of W 2 C NFs. Only electrochemical steps are shown. The parts of the reaction where chemical and electrochemical steps are essential are highlighted by colors. The favorable reactions of key chemical steps are provided (for free energies of these reactions, see Table S9 ). The intermediates are indicated. Gibbs free energies for reaction at zero potential vs RHE are given in eV. Full size image This pathway indicates that limiting steps (at zero potential with respect to RHE) are protonation of adsorbed CO 2 and O, and, most importantly, the desorption of H 2 O following protonation of adsorbed OH. The difficulty of this final step is not surprising, as W 2 C (101) strongly adsorbs and spontaneously dissociates water ( \({{{{{{\mathrm{H}}}}}}}_{2}{{{{{\mathrm{O}}}}}}\to {{{{{{\mathrm{H}}}}}}}^{\ast }+{{{{{{{\mathrm{OH}}}}}}}}^{\ast }\) , \(\triangle G=-1.797\,{eV}\) ) without electrochemical assistance. Similarly, our calculations indicate that W 2 C (101) strongly chemisorbs CO 2 ( \({{{{{{{\mathrm{CO}}}}}}}}_{2}\to {{{{{{{\mathrm{CO}}}}}}}}_{2}^{\ast },\triangle G=-1.24\,{eV}\) , bond length \(d\left(W-O\right)=2.04 \AA,{d}\left(W-C\right)=2.12 \AA\) ) in contrast to normally weak physisorption on Cu ( \(-0.3\,{eV}\) ) and other catalyst surfaces [28] , [67] , [68] , [69] . Furthermore, the (101) surface of W 2 C enables favorable and unassisted dissociation of adsorbed CO 2 ( \({{{{{{{\mathrm{CO}}}}}}}}_{2}^{\ast }\to {{{{{{{\mathrm{CO}}}}}}}}^{\ast }+{{{{{{\mathrm{O}}}}}}}^{\ast }\) , \(\triangle G=-0.97\,{eV}\) , Supplementary Table 10 ) suggesting that C–O bond scission may take place in the early stages of CO 2 reduction, skipping the uphill production of adsorbed carboxyl. Based on these findings, we propose that W 2 C (101) distinguishes itself as a catalyst due to an interplay between surface-assisted chemical steps, whose energetics will depend on the local chemical equilibrium at the surface and electrochemical steps that reduce preexisting surface reagents and open up new pathways for the overall reaction to proceed. More detailed studies of such cooperative catalytic processes and their limiting steps may be encouraged based on the promise of W 2 C as a high-performance CO 2 reduction catalyst. Here, we highlight the plausible cooperative effects of these steps, which set apart W 2 C from conventional noble metal catalysts and the other TMCs, specially for CH 4 production. The immediate benefit of the favorable chemical processes mentioned above should be a higher surface coverage of CO 2 (and consequently CO) and an excess of surface protons. This may explain the high Faradaic efficiencies for the production of both H 2 and CO at low potentials (see Supplementary section 3 and Supplementary Table 1 ). However, once a limiting potential (−0.74 V estimate) is reached, the readily protonated products of adsorbed CO that produce CH 4 are no longer hindered by a build-up of adsorbed byproducts (O* then OH*), which can now be protonated and released from the surface. We can divide the complex, multistep reaction into two key parts: initial conversion of adsorbed CO 2 to adsorbed CO, followed by conversion of adsorbed CO to CH 4 with the release of H 2 O (see Fig. 3 and Supplementary Fig. 27 ). As indicated in Fig. 3 , the first part, generation of adsorbed CO, can be achieved by chemical or electrochemical means. We have direct and favorable chemical conversion of adsorbed CO 2 to adsorbed CO and O on W 2 C (101), but also two electrochemical pathways: production of HO–CO* in a single step (+0.66 eV, Fig. 3 ) or an alternative initially favorable protonation to OCHO* followed by two uphill electrochemical steps producing the first OCH 2 O* followed by the release of H 2 and the final product of HO–CO* with a similar free energy cost (+0.68 eV, Supplementary Fig. 27 and Supplementary Table 10 ). A final electrochemically driven protonation of HO–CO* favorably releases H 2 O and leaves CO*. With chemically or electrochemically generated adsorbed CO, we can proceed to the second part of the overall reaction to produce CH 4 from CO 2 , which involves multiple favorable protonation steps. The W 2 C catalyst distinguishes itself here. The electrochemical activation of \({{{{{{{\mathrm{CO}}}}}}}}^{\ast }\to {{{{{{{\mathrm{HCO}}}}}}}}^{\ast }\) remains thermodynamically favorable (ΔG = −0.26 eV) on W 2 C (101), whereas on other catalysts, such as Cu, this process is usually uphill with the potential ranging from −0.74 to −0.97 V vs RHE [66] , [70] . Moreover, due to the spontaneous water dissociation, the direct H* transfer step \({{{{{{{\mathrm{CO}}}}}}}}^{\ast }+{{{{{{\mathrm{H}}}}}}}^{\ast }\to {{{{{{{\mathrm{HCO}}}}}}}}^{\ast }\) on W 2 C could be even more favorable with a resultant ΔG = −0.433 eV (Supplementary Table 10 ). The next two electrochemical steps are downhill (ΔG = −0.04 and −0.58 eV): the first forming the unstable methoxy radical \({{{{{{\mathrm{C}}}}}}{{{{{{\mathrm{H}}}}}}}_{3}{{{{{\mathrm{O}}}}}}}^{\ast }\) with oxygen attached to a surface W atom; the second leading to spontaneous dissociation into the methyl radical \({{{{{{{\mathrm{CH}}}}}}}}_{3}^{\ast }\) and a surface oxygen atom \({{{{{{\mathrm{O}}}}}}}^{\ast }\) . The electrochemical conversion of the surface \({{{{{{{\mathrm{CH}}}}}}}}_{3}^{\ast }\) into CH 4 is favorable (ΔG = −0.43 eV) and the protonation of the surface oxygen \({{{{{{\mathrm{O}}}}}}}^{\ast }\) is only slightly uphill (ΔG = +0.03 eV). As we already stated, for the overall reaction \({{{{{\mathrm{C}}}}}}{{{{{{\mathrm{O}}}}}}}_{2}^{\ast }+8{{{{{{\mathrm{H}}}}}}}^{+}/{{e}}^{-}\to \ast +2{{{{{{\mathrm{H}}}}}}}_{2}{{{{{\mathrm{O}}}}}}+{{{{{{{\mathrm{CH}}}}}}}}_{4}\) on W 2 C (101) it is the final protonation of \({{{{{{\mathrm{OH}}}}}}}^{\ast }\) to release H 2 O that is the limiting step (ΔG = +0.74 eV). We also compared W 2 C with the other TMCs studied by calculating the energies of adsorption of water and CO 2 as well as the potentials of the rate-determining step (i.e., protonation of \({{{{{{{\mathrm{OH}}}}}}}}^{\ast }\) ) for Nb 2 C, Mo 2 C, and V 2 C (Supplementary Table 11 ). Our calculations indicate that these TMCs also strongly chemisorb CO 2 with adsorption energies of −1.32, −1.62, and −0.96 eV, respectively. Moreover, Nb 2 C also shows favorable C–O bond scission of adsorbed CO 2 . Additionally, Nb 2 C, Mo 2 C, and V 2 C strongly adsorb water with the energies of −1.87, −1.23, and −0.59 eV, respectively, where Nb 2 C is the only other catalyst that dissociates water. In contrast to W 2 C, the energies required for the protonation of \({{{{{{{\mathrm{OH}}}}}}}}^{\ast }\) are higher: +1.17, +1.25, and +0.85 eV for Nb 2 C, Mo 2 C, and V 2 C, respectively (Supplementary Table 11 ). Therefore, we can conclude that, within this set of four TMCs, W 2 C possesses the optimal characteristics for efficient completion of CO 2 RR: (1) sufficiently strong adsorption of CO 2 , (2) spontaneous dissociation of water, and (3) the lowest limiting potential for OH* protonation. We conclude that the performance of Nb 2 C is reduced due to its stronger water adsorption, resulting in the protonation of \({{{{{{{\mathrm{OH}}}}}}}}^{\ast }\) requiring more energy. We would expect Mo 2 C to have a lower surface coverage of protons and higher costs for the protonation of \({{{{{{{\mathrm{OH}}}}}}}}^{\ast }\) . The weakest CO 2 adsorption on V 2 C decreases its surface coverage, making it the worst TMC catalyst here, despite its relatively small limiting reaction potential of protonation of OH*. As we mentioned before, for W 2 C the realistic network of pathways towards CH 4 consists of a potential-dependent combination of competing chemical and electrochemical steps with the actual limiting potential being in the range from −0.483 to −0.744 V vs RHE (see the full path. Supplementary Fig. 27 ), which is consistent with our three-electrode electrochemical experimental results (Supplementary section 3 and Supplementary Table 1 ). A steeper Tafel slope for CH 4 formation on W 2 C than other TMCs and Cu, (Supplementary Fig. 8 ) also indicates the competition between reactions for the active sites on the catalyst surface. Specifically, the spontaneous water dissociation on W 2 C (101) explains the ease of the HER in our nonacidic electrolyte where the source of protons is normally water. A weak potential dependence of the partial CO current and its small overpotential also originate from the interplay between chemical and electrochemical steps (see Supplementary Information for details). Experimentally, we have studied the effect of CC on the activity and selectivity of the TMC catalysts. To do this, we have performed electrochemical CO 2 RR in different CC concentrations of i.e., 0.01, 0.1, 1, and 2 M mixed with 3 M KOH (Supplementary section 14 ). 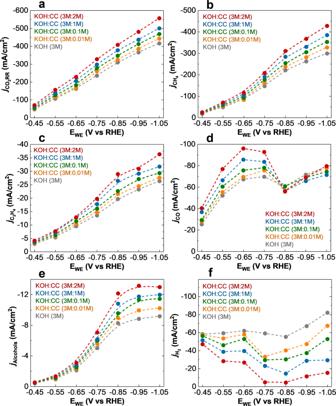Fig. 4: Effect of choline chloride in the electrochemical performance of W2C NFs for CO2RR. The values are measured using 3 M KOH and mixed 3 M KOH with different concentrations (0.1, 0.01, 1, and 2 M) of choline chloride (CC) electrolytes. Partial current density (j) measurements foraCO2RR,bCH4,cC2H4,dCO,eAlcohols (CH3OH and C2H5OH), andfH2as a function of potential (EWE). Figure 4 shows CO 2 RR overall current density and different products (i.e., CH 4 , C 2 H 4 , CO, alcohols-CH 3 OH, and C 2 H 5 OH- and H 2 ) partial current densities for W 2 C NFs in different CC concentration electrolytes. Figure 4a indicates that by increasing the concentration of CC in the electrolyte the CO 2 RR current density ( j CO2RR ) increases and reaches a maximum value of −548.89 mA/cm 2 at a potential of −1.05 V vs RHE for 2 M of CC. The obtained value is about 32, 24, and 17, 9% higher than that of 0, 0.01, 0.1, and 1 M of CC, respectively. Moreover, a maximum CH 4 formation current density ( j CH4 ) of −421.63 mA/cm 2 is obtained for 2 M CC at a potential of −1.05 V vs RHE that is about 1.41, 1.29, 1.19, and 1.1 times higher than that of 0, 0.01, 0.1, and 1 M, respectively (Fig. 4b ). Fig. 4: Effect of choline chloride in the electrochemical performance of W 2 C NFs for CO 2 RR. The values are measured using 3 M KOH and mixed 3 M KOH with different concentrations (0.1, 0.01, 1, and 2 M) of choline chloride (CC) electrolytes. Partial current density ( j ) measurements for a CO 2 RR, b CH 4 , c C 2 H 4 , d CO, e Alcohols (CH 3 OH and C 2 H 5 OH), and f H 2 as a function of potential (E WE ). Full size image The results also indicate using W 2 C NFs, maximum partial current densities of other products i.e., C 2 H 4 ( j C2H4 of −35.84 mA/cm 2 ), CO ( j CO of −78.48 mA/cm 2 ), and alcohols ( j Alcohols of −12.81 mA/cm 2 ; −6.84 mA/cm 2 for CH 3 OH and −5.97 mA/cm 2 for C 2 H 5 OH) were obtained at the potential of −1.05 V vs RHE in 2 M CC (Fig. 4b–d ). In contrast, the measured H 2 partial current densities indicate that by adding a higher concentration of CC to the electrolyte solution the rate of H 2 production decreases significantly where a minimum H 2 formation current density of −4.48 mA/cm 2 was obtained for 2 M CC at a potential of −0.85 V vs RHE that is 12.31, 8.97, 6.76, 3.23 times lower than that of 0, 0.01, 0.1 and 1 M CC, respectively. These results suggest that adding CC to the 3 M KOH electrolyte suppresses the competing HER and increases the formation of CO 2 RR products more specifically CH 4 [27] . The stability of the CC electrolytes was studied by conducting nuclear magnetic resonance (NMR) and 13 CO 2 isotope experiments (Supplementary sections15 and 16 ) [27] , [46] , [71] . The 1 H and 13 C NMR spectra reveal similar peak areas and chemical shifts for fresh and used electrolytes indicating no generation of new diamagnetic species or change in the CC structure under an applied potential of −1.05 V vs RHE (Supplementary Figs. 38 , 39 ). The 13 CO 2 isotope experiments also show that the CO 2 gas present inside the electrolyte is the only source of the formed products in the electrochemical CO 2 RR (Supplementary Fig. 41 ). These results confirm that CC with different concentrations i.e., 0, 01, 0.1, 1, and 2M remains stable at the range of applied potentials in the electrochemical CO 2 RR experiments. Next, we studied the performance of W 2 C NFs in our developed solid polymer electrolyte flow electrolyzer for continuous electrochemical CO 2 RR using this catalyst as the cathode (Supplementary section 17 ). The flow electrolyzer used in this study consists of a two-compartment electrochemical setup with an active area of 5 cm 2 coated with W 2 C NFs at the cathode and iridium oxide nanoparticles (IrO 2 NPs) as the anode and were then fed with humidified CO 2 and KOH:CC (3 M:2 M) electrolyte, respectively (Supplementary section 17 ). To study the CO 2 RR performance of W 2 C NFs in the flow electrolyzer, we performed chronoamperometry (CA) experiments at different cell potentials ranging from −1.5 to −2.3 V for W 2 C NFs (Supplementary section 17 ). As shown in Fig. 5a , the results show that at a cell potential of −1.5 V, hydrogen (H 2 , FE of 54.9% ± 1.4) and CO (FE of 40.1% ± 1.8) are the dominant products. However, our measurements indicate that by increasing the cell potential a system becomes more selective for CH 4 formation with the maximum FE of 82.7% ± 2 at a cell potential of −2.1 V. At this potential, W 2 C NFs slightly produce other products such as C 2 H 4 , CH 3 OH, C 2 H 5 OH, CO, and H 2 with FEs of 5.6, 1.4, 1.2, 6.1, and 1.4, respectively. 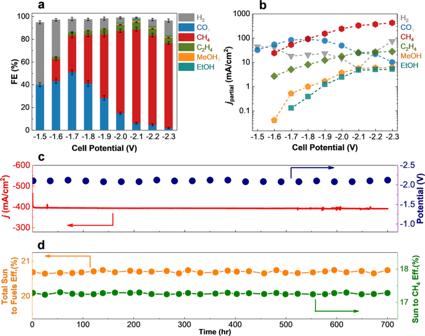Fig. 5: Electrocatalytic performance and stability of W2C NFs in the solid polymer electrolyte flow electrolyzer. aFaradaic efficiency (FE) measurements of H2, CO, CH4, C2H4, methanol (MeOH), and ethanol (EtOH) for W2C NFs at different cell potentials. The error bars represent standard deviations of four independent experiments.bPartial current density for each product as a function of cell potential. The values are obtained considering the total current density and faradaic efficiencies of products at the entire range of cell potential.cMeasured total current densities and cell potentials of the solar-driven solid polymer electrolyte flow electrolyzer under one sun illumination provided by the TJ-PV cell over time.dTotal sun to fuels efficiency and sun to CH4production efficiency in the solar-driven solid polymer electrolyte flow electrolyzer over time. Figure 5b shows the maximum CH 4 , C 2 H 4 , CH 3 OH, and C 2 H 5 OH current densities of −421.28, −27.31, −5.95, and −5.19 mA/cm 2 at the cell potential of −2.3 V, respectively, confirming high selectivity of W 2 C NFs towards CH 4 as the main product. Fig. 5: Electrocatalytic performance and stability of W 2 C NFs in the solid polymer electrolyte flow electrolyzer. a Faradaic efficiency (FE) measurements of H 2 , CO, CH 4 , C 2 H 4 , methanol (MeOH), and ethanol (EtOH) for W 2 C NFs at different cell potentials. The error bars represent standard deviations of four independent experiments. b Partial current density for each product as a function of cell potential. The values are obtained considering the total current density and faradaic efficiencies of products at the entire range of cell potential. c Measured total current densities and cell potentials of the solar-driven solid polymer electrolyte flow electrolyzer under one sun illumination provided by the TJ-PV cell over time. d Total sun to fuels efficiency and sun to CH 4 production efficiency in the solar-driven solid polymer electrolyte flow electrolyzer over time. Full size image Next, we coupled the electrolyzer to a triple junction photovoltaic (TJ-PV) cell with a maximum efficiency of 34.3% to determine the CO 2 RR performance and energy efficiency of W 2 C NFs in a solar-driven device (Supplementary section 18 ). The j-V characteristic curve of the TJ-PV cell under one sun illumination (100 mW/cm 2 ) using a sun simulator light source is shown in Supplementary Fig. 48 . The operating point is chosen to provide a photocurrent density of −394.3 mA/cm 2 at a potential of −2.1 V which has the maximum FE of CH 4 (82.7% ± 2) calculated in the flow electrolyzer (Supplementary Fig. 49 ). Figure 5c shows the current density of the solar-driven electrolyzer for a 700-h continuous process at a potential of −2.1 V. The results shown in Fig. 5c indicate a negligible decrease (~2%) in the photocurrent density of W 2 C NFs over the 700-h experiment while the corresponding photo-potential fluctuates between −2.08 to −2.12 V, confirming the high stability of W 2 C NFs for CO 2 RR. The measured sun to CO 2 RR products (CO, CH 4 , C 2 H 4 , CH 3 OH, and C 2 H 5 OH) as well as total solar-to-fuel efficiency (SFE) of W 2 C NFs over a 700-h process are shown in Fig. 5d (Supplementary section 18 ). As shown in this figure, an average sun to the CH 4 production efficiency of 17.3% with negligible variation (2%) is achieved during the 700-h continuous process. Considering other products, W 2 C NFs show an SFE of 20.7%. We also calculated the energy efficiency of CO 2 RR in our developed flow electrolyzer and compared it with state-of-the-art catalytic systems in the literature (Supplementary section 17 ) [29] , [30] , [37] , [57] , [72] . As shown in this figure (Supplementary Fig. 47 ), the maximum energy efficiency of 62.3% was obtained for our developed flow electrolyzer using W 2 C catalyst that is about 67 and 73% more efficient than Cu oh (37.4%) [50] and recently developed Cu-CIPH (36.1%) [72] catalytic systems, respectively. In summary, we have synthesized four members of TMCs with a formula of M 2 C, i.e., W 2 C, Mo 2 C, Nb 2 C, and V 2 C NFs using the carburization method followed by the liquid exfoliation technique and tested their catalytic performance for eCO 2 RR in KOH:CC (3 M:2 M) electrolyte. The electrocatalytic performance studies of TMCs shows these materials are mainly selective for CH 4 formation with W 2 C NFs having the best CO 2 RR activity compared to the studied catalysts. For instance, a CO 2 RR current density of −548.89 mA/cm 2 and a maximum CH 4 current density of −421.63 mA/cm 2 at the potential of −1.05 V vs RHE were observed for W 2 C NFs. Our electrochemical results also indicate that adding CC to the electrolyte enhances the formation of CO 2 RR products by suppressing the HER for all studied TMCs. Moreover, the NMR and 13 CO 2 isotope experiments confirm that the CC remains stable during the electrochemical experiments. Atomic and molecular scale characterizations such as XPS, XRD, and STEM indicate that all synthesized TMCs have a similar lattice structure of 1 T with a dominant plane of (101) and almost the same average crystallite size of 25.4 nm. Furthermore, the electronic property analyses of TMCs reveal superior electronic properties of W 2 C NFs: low work function; small charge transfer resistance in the electrochemical double layer region; and heavily reduced tungsten atoms at the surface, which may lead to the observed high activity. Computational results also indicate that the studied TMCs spontaneously chemisorb CO 2 and water as compared to Cu. However, among the TMCs studied, W 2 C exhibits the optimal combination for CH 4 production, with favorable adsorption energies of water and CO 2 coupled with spontaneous dissociation, and less costly protonation of OH*, which is the limiting step, with a low limiting potential in the range of −0.483 to −0.744 V vs RHE. Using W 2 C NFs, we have demonstrated a solar-driven flow electrolyzer that can work up to 700 h with a solar to CH 4 efficiency and a total SFE of 17.3 and 20.7%, respectively, under one sun illumination. The demonstrated solar-driven flow electrolyzer using a non-precious metal catalyst (W 2 C NFs) in this study achieves maximum efficiency of 62.3% making it a good candidate to approach the commercially relevant electrocatalytic CO 2 RR. This opens a new direction toward a low-cost, sustainable large-scale production of fuels from CO 2 that can be used any time any place. Synthesis of TMCs TMCs were prepared by carburization process in a dual-zone tubular furnace with a controlled flow of CH 4 and H 2 mixture (volumetric ratio CH 4 :H 2 of 1:9) at a temperature of 973 K. The obtained bulk powders were then collected and ground to fine powders in a mortar and pestle. Next, a certain amount of TMC powders were processed in isopropyl alcohol using an ultrasonic liquid processor (Sonics VibraCell VCX-130) to obtain a solution of TMC NFs. The resulting solution was further centrifuged and the top two-third of the solutions were collected and stored as the TMCs in a vial for cathode electrode preparation. A detailed explanation is provided in Supplementary section 1 . Electrochemical setup A two-compartment three-electrode electrochemical cell was used to perform the fundamental study for cathodic half-cell reaction using the synthesized W 2 C, Mo 2 C, Nb 2 C, and V 2 C NFs and compared them with Au and Cu NPs. In the three-electrode cell study, the working electrode was prepared by drop-casting the catalysts (mass loading of 0.1 mg) on a glassy carbon electrode with a geometric surface area of 1 cm 2 . The catalyst loading on the electrode was precisely controlled to be 0.1 mg/cm 2 on the glassy carbon electrode. Platinum (Pt) gauze 52 mesh (Alfa Aesar) and Ag/AgCl (BASi) were used as counter and reference electrodes, respectively. The cathode and anode parts of the cell were separated through an anion exchange membrane (Sustainion X37-50 Grade RT, Dioxide Materials). All experiments were performed in a CO 2 saturated KOH:CC (3 M:2 M) electrolyte with a pH of 14.5 ± 0.1. A two-compartment zero-gap solid polymer electrolyte flow electrolyzer was used to study the electrochemical performance where the working and counter electrodes are separated using an anion exchange membrane. Working electrodes (cathode) were prepared by brush-coating the solution of studied catalysts (W 2 C NFs, Au NPs, and Cu NPs) on the gas diffusion layer (GDL, Sigracet 39 BC, Fuel Cell Store) electrodes with a geometrical surface area of 5 cm 2 . The counter electrode (anode) was prepared using a similar procedure where IrO 2 powder (Sigma Aldrich) was used as the catalyst solution. The actual loadings of 0.1 ± 0.01 mg/cm 2 were determined by weighing the dry GDLs before catalyst deposition and coated GDLs after being dried in a vacuum oven overnight. As a separator in our experiments, we used an anion exchange membrane (Sustainion X37-50 Grade RT, Dioxide Materials) which was treated in 1 M KOH overnight at 75 °C and then washed with deionized water prior to use. Anolyte flow of KOH:CC (3 M:2 M) with a flow rate of 20 ml/min was fed to the anode compartment using a peristaltic pump (Masterflex, Cole-Parmer). A mass flow controller (SmartTrak 50, Sierra, calibrated with CO 2 gas) connected to the CO 2 humidifier kit, was used to feed the cathode compartment with a flow rate of 50 ml/min. PV cell characterization A solar-powered flow cell was assembled by connecting the solid polymer electrolyte flow electrolyzer to a triple junction photovoltaic (TJ-PV) solar cell. The TJ-PV cell was characterized at different sun illuminations using a custom-made sun simulator light source and an InGaAs photodiode (Thorlabs, FDG03-CAL) with a known responsivity calibration curve. Our results indicated a maximum efficiency of 34.32% under one sun illumination used in our study. Electrochemical characterization Electrochemical experiments were performed using a Biologic Potentiostat SP-150. The CA technique was used to study the performance of TMC NFs i.e., W 2 C, Mo 2 C, Nb 2 C, and V 2 C NFs and compared them with that of Au and Cu NPs. The CA experiments were carried out in the range of −0.45 to −1.05 V vs RHE potentials. All experiments were performed under identical experimental conditions. The LSV technique was used to study the fundamentals of the cathodic half-cell reaction in the three-electrode cell setup. LSV curves were obtained by sweeping the potential between +0.2 and −1.05 V vs RHE with a scan rate of 20 mV/s. The conversion of Ag/AgCl reference electrode potential to the RHE scale was calculated using the Nernst equation considering the pH of the solution (pH = 14.5). Product characterization A gas chromatography system (GC, SRI, 8610 C) equipped with a flame ionization detector (FID) and a thermal conductivity detector (TCD) was used to detect and quantify the electrochemical CO 2 RR products. Ultra-high purity helium (He) and nitrogen (N 2 ) gases (UHP 99.99%, Airgas) were used as the carrier gas to identify any possible type of product. the signal response of the FID and TCD to each gaseous product (e.g., H 2 , CO, CH 4 , and C 2 H 4 ) was calibrated by analyzing a series of standard gas mixtures with known compositions prior to the experiments. To study the products, 1 mL sample of the headspace of the cell was injected into the GC system using a lock-in syringe (Hamilton). Moreover, an in situ differential electrochemical mass spectrometer (DEMS, Hiden Analytical, HPR-40) was used to validate the obtained information from the GC system by continuously detecting all possible products, even at trace amounts (partial pressure of 1 × 10 −13 Torr), during the electrochemical CO 2 RR (CA experiment), resulting in more precise measurement. The signal responses of the DEMS instrument for different products (H 2 , CO, CH 4 , C 2 H 4 , CH 3 OH, and C 2 H 5 OH) were calibrated by feeding standard samples into the mass spectrometer. An electron energy of 70 eV was used for ionization of all species, with an emission current of 500 µA. All mass-selected product cations were detected by a secondary electron multiplier with a detector voltage of 1200 V for maximizing the signal-to-noise ratio of the products. X-ray diffraction (XRD) The XRD technique was used to identify the phase purity and crystallinity of all studied catalysts (W 2 C, Mo 2 C, Nb 2 C, V 2 C NFs, Au NPs, and Cu NPs) using a Bruker D2 PHASER diffractometer in Bragg–Brentano geometry employing a Ni filtered Cu K α radiation (1.5405 Å). The XRD patterns were obtained using a LynxEye linear position-sensitive detector and a step width of 0.2 °2θ with a counting time of 1 s/step. X-ray photoelectron spectroscopy (XPS) A Thermo-Scientific ESCALAB 250Xi instrument equipped with an electron flood and scanning ion gun was used to identify the oxidation states of the W 2 C NFs. All obtained spectra were analyzed using Thermo-Avantage software, considering the standard carbon peak at 284.8 eV and relative sensitivity factors. Ultraviolet photoelectron spectroscopy (UPS) Surface work function measurements were carried out using the UPS technique. All UPS data were acquired by a Thermo-Scientific ESCALAB 250Xi instrument using He I (21.2 eV) ultraviolet radiation and a pass energy of 8.95 eV. Scanning transmission electron microscopy (STEM) W 2 C NFs were characterized at the atomic scale using a spherical aberration-corrected JEOL JEM-ARM 200CF STEM with a cold field emission gun operating at 200 kV. HAADF detector with 22 mrd inner-detector angle and BF detector were utilized to obtain the atomic resolution images. Theoretical study We performed a comparative DFT analysis for the observed catalytic activity and reactivity of W 2 C NFs with Au and other TMCs using the SIESTA package, with Perdew–Burke–Ernzerhof functional with a double-zeta with polarization (DZP) localized basis set and the norm-conserving Troullier-Martins pseudopotentials. Calculations of DOS for bulk and slab geometries of Au and TMCs were performed using the Effective Screening Method (ESM) [73] for Brillouin zones of the unit cells sampled by Monkhorst-Pack k-point grids of size 9 × 9 × 9 and 1 × 9 × 9, respectively, together with a plane-wave cutoff of 300.0 Ry. The optimization of the atomic positions and cell parameters were carried out using a conjugate-gradient algorithm until a maximum atomic force tolerance of 0.04 eV/Å and a maximum stress component along each periodic direction of lower than 1 GPa were achieved. The Vienna ab initio Simulation Package (VASP, version 5.4.4) with PAW (projector augmented wave method) and Perdew–Burke–Ernzerhof exchange-correlation functionals were used to analyze the adsorption free energies of various molecular species on the (101) surface of M 2 C (M = W, V, Mo, Nb). All the VASP calculations were performed for neutral non-spin-polarized systems and a dipolar electrostatic correction was used along the normal to the surface of the slab. Next, we used the tetrahedron method with Blöchl corrections and 1 × 3 x 3 Monkhorst-Pack grid k-point sampling for the calculations of total electronic energy (smearing σ = 0.1). The adsorption free energies were then used within the CHE model [64] , [65] , [66] to evaluate the lowest free energy pathways and the limiting reaction potentials.